Long-term experimental hybridisation results in the evolution of a new sex chromosome in swordtail fish The remarkable diversity of sex determination mechanisms known in fish may be fuelled by exceptionally high rates of sex chromosome turnovers or transitions. However, the evolutionary causes and genomic mechanisms underlying this variation and instability are yet to be understood. Here we report on an over 30-year evolutionary experiment in which we tested the genomic consequences of hybridisation and selection between two Xiphophorus fish species with different sex chromosome systems. We find that introgression and imposing selection for pigmentation phenotypes results in the retention of an unexpectedly large maternally derived genomic region. During the hybridisation process, the sex-determining region of the X chromosome from one parental species was translocated to an autosome in the hybrids leading to the evolution of a new sex chromosome. Our results highlight the complexity of factors contributing to patterns observed in hybrid genomes, and we experimentally demonstrate that hybridisation can catalyze rapid evolution of a new sex chromosome. Sex chromosomes evolve from autosomes and are typically extremely conserved, not only among species but entire classes of organisms. The best-studied sex chromosome systems are ZW and XY, female and male heterogametic systems respectively. These categorical sex-determining systems have evolved repeatedly and independently in the animal and plant kingdoms [1] . Yet genomic studies have also revealed several examples of rapidly evolving sex-determining mechanisms in closely related species of fish [2] , [3] , [4] , [5] , [6] , [7] , and also in amphibians [8] , [9] and reptiles [10] , [11] . Even between sister taxa of fishes, instances are known where either males or females are heterogametic. However, despite much theoretical work and empirical findings of convergent evolution of sex chromosomes [11] , [12] , [13] , [14] , [15] , [16] , why such variety in something as fundamental as the mechanisms of sex determination exists, and how it evolves, remains elusive. If two closely related lineages differ in their sex chromosome systems, several scenarios for the emergence of this difference are possible [17] : either there was no chromosomal sex determination in the last common ancestor and both systems developed independently, or one lineage retained the ancestral sex chromosomes while in the other lineage a transition to the alternate system occurred. Theoretically, such transitions can happen on the same pair of sex chromosomes (homologous transition) or involve an autosome, which then becomes a new sex chromosome (heterologous transition). At the molecular level, the gene(s) determining sex might have changed their mode of action, e.g. from female to male determination, or a novel sex-determining (SD) gene might have arisen and taken over (SD turnover) in the evolving lineage. An intriguing scenario in sex chromosome evolution connected to speciation is hybridisation, particularly in crosses of species with different male and female heterogametic sex chromosomes. Based on Haldane’s rule, one would expect that the heterogametic sex in hybrids tends to show greater inviability or sterility than the homogametic sex [18] and one proposed explanation for this is dominance theory [19] . Hybrids between different species might be expected to suffer deleterious incompatibilities because alleles from orthologous genes from different species may not interact well in hybrids, and if these genes are on the sex chromosomes and are recessive, the heterogametic sex is likely to suffer the most. This would be expected to result in selection for alternative sex chromosome systems in lineages arising from a hybridisation event. As intriguing as these concepts are, empirical evidence for the evolution of new sex chromosome systems following hybridization is very scant because these events have happened in the evolutionary past and would be expected to take long time periods to complete. Still, in some laboratory animals the loss of a sex-determining locus has been observed (e.g. medaka [20] and zebrafish [21] ), but these domesticated lines have not yet developed a new stable mechanism of the same kind (a sex determination turnover) or completed a transition. In vertebrates, teleost fish show an enormous diversity of sex chromosome systems, hence turnovers or transitions must have occurred more often than in most other classes of vertebrates (e.g. ref. [7] ). Therefore, the study of closely related species of fishes that exhibit different sex chromosome systems would be particularly informative for the investigation of the evolution of mechanisms of sex determination (e.g. ref. [7] ). Among the 26 species of the genus Xiphophorus (swordtails and platyfish) are species with both XY and ZW sex chromosome systems [22] , [23] . In this genus, these simple heterogametic systems are both present together with more complex situations that can include multiple loci and chromosomes [23] , [24] . Xiphophorus maculatus , for example, one of the most well studied and geographically widespread species in this genus, has three different genetically well-defined sex chromosomes, X, Y and W. Possible female genotypes are XX, XW and YW, and in males XY or YY. Several different models have been proposed to explain sex determination with three sex chromosomes in this species [25] , [26] . While in the wild in most populations all these sex chromosome combinations co-exist, laboratory lines have been established which are stable for XY/XX or WY/YY sex determination. WW females can be generated in the laboratory after experimental manipulation and are viable, but such individuals have not been reported in natural populations [23] . In several species, autosomal modifiers, which occur at low frequency in natural populations, have also been reported to act, and may explain instances of atypical sex determination [24] , [25] . As another example of sex determination variation in this genus, in Xiphophorus hellerii, a polyfactorial sex-determining system has been reported to be acting. Additionally, it has been suggested that this species has a main genetic system affected by numerous autosomal modifiers, while more recent studies report that some strains of X. hellerii have a XW–YY female heterogametic system [22] , [23] . To our knowledge, environmental sex determination has not been reported from observations in nature or from laboratory studies in the genus Xiphophorus . In general, this genus of fish comprises well known and widely studied models for organismic and molecular evolution. In particular, Xiphophorus species have been used as a model system for studying the evolutionary genetics of hybridisation for more than 50 years [27] , [28] , [29] , [30] , [31] , [32] with a recent resurgence of investigations using modern molecular and genomic data [27] , [33] , [34] , [35] , [36] , [37] , [38] . Ancient hybridisation events between many species in this genus has been inferred [27] , [36] , [37] , [39] and may be facilitated by apparently weak postzygotic isolation in Xiphophorus [39] , [40] , [41] . We previously utilized SNP data from RAD sequencing to estimate the phylogenetic relationships among all 26 Xiphophorus species, and uncovered incongruence between the RAD-nuclear vs. mtDNA phylogenies [33] , [36] , [42] . This phylogenetic incongruence likely reflects the contribution of hybridisation to the evolution of two Xiphophorus species ( Xiphophorus clemenciae and Xiphophorus monticolus) [36] . Such phylogenetic incongruence, in addition to asymmetrical behavioural preferences of first generation hybrids and the morphology of the putative hybrid taxon being much closer to one of the possible parental species [33] , provides support for hybridisation followed by repeated backcrossing having contributed to the evolution of these species. The inferred ancient hybridisation event likely involved a female Southern platyfish, X. maculatus , and a male green swordtail, X. hellerii . Evidence for reticulate evolution is typically inferred from analyses of extant populations or species. However, the actual processes contributing to the introduction of an allospecific genome and the fate of the extra-specific genetic material are difficult to identify and document. To better understand the genomic consequences of interspecific hybridisation for sex chromosome evolution and speciation, we conducted a long-term crossing experiment (conducted for >30 years and spanning >100 generations) in fish of the genus Xiphophorus (Fig. 1 ). We experimentally mimic the evolutionary scenario, hybridisation with repeated backcrossing, which is thought to have contributed to the evolution of at least two of the 26 species in the genus Xiphophorus [33] , [36] , [37] . Of particular interest is that the parental species used in the experimental evolutionary crosses differ in their sex chromosome systems. The maternal lineage used here, the platyfish X. maculatus Jp163A strain, has an XY sex chromosome system [43] , whereas the backcross paternal lineage, the swordtail X. hellerii strain originating in the Rio Lancetilla, has a ZW sex chromosome system. This experimental set up enabled us to investigate the genomic consequences of known hybrid ancestry and timing, and specifically the consequences of sex chromosome evolution. We find that during the process of continuous introgressive breeding, the sex-determining region of the X chromosome derived from the maternal ancestor was translocated to an autosome of the receiving genome, thus providing empirical experimental evidence of a heterologous transition. We also note that at its new chromosomal position the former X-chromosome-specific region is located in a large region of retained maternal sequences, indicating that the loss of recombination accompanied the establishment of the novel W chromosome. Fig. 1 Schematic outline of the laboratory cross. The parental species X. maculatus and X. hellerii , a female specimen of the first generation hybrid and the resulting offspring obtained after approximately 100 generation of backcrosses (see Methods for details) are shown. The dorsal red ( Dr ), the spotted dorsal ( Sd ) and the oncogene xmrk loci, closely linked on the X-chromosome of the platyfish (LG21), are also highlighted. A translocation event of a genomic region containing these loci accompanied by recombination suppression has likely contributed to the formation of a new sex chromosome, a neo W chromosome (LG2), during the backcross experiment. Fish images by M. Schartl Full size image Identification of the sex-determining system and sex linkage group in X. hellerii The sex determination system of the platyfish strain used for our study is firmly established as XY, not only from a plethora of crossing data but also from molecular genetic evidence, and there is no evidence for an influence of autosomal or environmental modifiers (e.g. the platyfish genome was based on the same strain [43] ). However, for X. hellerii the situation is less clear and there are conflicting reports ranging from pure ZW heterogamety to a polyfactorial system with the absence of sex chromosomes [44] , [45] . To identify the sex-determining (SD) system in X. hellerii , deep coverage RAD sequencing of 60 X. hellerii individuals (30 males and 30 females) of the Rio Lancetilla strain was done (sequencing statistics for each individual is provided in Supplementary Data 1 ). To identify genomic regions associated with sex in X. hellerii , we employed a genome-wide association study (GWAS) and an analysis of genetic differentiation (F ST ). For these analyses, we used the X. maculatus v4.4.2 as the reference genome [46] , where the sex chromosome pair was clearly detected in linkage group 21 (LG21). Given the high level of synteny conservation between the two species’ genomes [47] this approach allowed us to directly compare the sex chromosome regions of X. maculatus and X. hellerii by plotting the GWAS p -values and the F ST estimates on the X. maculatus linkage groups. The GWAS approach identified a large genomic region strongly associated with sex distal on LG21, spanning more than 1/3 of the LG (a genomic region of approximately 10 Mb, from ~13 to ~23 Mb, at the end of LG21) (Fig. 2b ). This region includes 243 SNPs that exceeded the Bonferroni-corrected genome-wide threshold ( p -value = 7.64e −7 ) and showed an excess of heterozygosity in females vs. males, conforming to expectations under a ZW sex determination system. A weaker association was identified in LG7, where 15 SNPs exceeded a threshold suggestive of significance ( p < 0.0001) (the location of the SNPs highly associated with sex that exceed the thresholds are shown in Supplementary Data 2 ). A second region of increased female sex linked heterozygosity besides LG21 representing the W/Z pair was unexpected. A reasonable explanation is that this region may play a role as a minor sex modifier. Such autosomal modifiers of a major sex chromosomal system have frequently been noted in the genus Xiphophorus [24] . 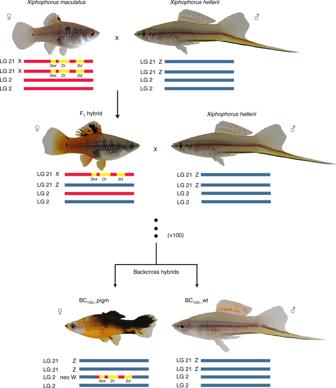Fig. 1 Schematic outline of the laboratory cross. The parental speciesX. maculatusandX. hellerii, a female specimen of the first generation hybrid and the resulting offspring obtained after approximately 100 generation of backcrosses (see Methods for details) are shown. Thedorsal red(Dr), thespotted dorsal(Sd) and the oncogenexmrkloci, closely linked on the X-chromosome of the platyfish (LG21), are also highlighted. A translocation event of a genomic region containing these loci accompanied by recombination suppression has likely contributed to the formation of a new sex chromosome, a neo W chromosome (LG2), during the backcross experiment. Fish images by M. Schartl Further, in our laboratory cross experiments (see below) we observed exceptional cases of males with a BC 100 _pigm phenotype and females with a BC 100 _wt phenotype (Supplementary Table 1 ). Such cases may be caused by autosomal modifiers. Fig. 2 Sex-determination system in Xiphophorus hellerii . a A male and female specimen of X. hellerii , males are clearly distinguished by the elongated caudal fin, ‘the sword’ (Fish images by M. Schartl). b Genome-wide association analysis, where sex is set as a binary case/control variable. The 65,417 SNPs that passed quality control were used in this analysis. The Manhattan plot shows the −log 10 p -value (Fisher’s exact test) of each SNP across the 24 X. maculatus linkage groups (LGs). The dashed red line indicates the genome-wide significance level ( p -value = 7.79e −7 ), while a suggestive significance ( p -value = 0.001) is denoted by the dashed black line. Orange and blue colours are used to distinguish between LGs. The peak showing the strongest association is located on LG21, and is enlarged in the bottom-right section of the panel. c Sequence coverage of RAD loci in female and male X. hellerii individuals. Each dot in the scatter plot represents the average coverage across all males ( x -axis) against the average coverage across all females ( y -axis) for each of the selected RAD loci. Red dots indicate potential W-linked loci (female-specific loci), while blue dots indicate loci potentially linked to the Z chromosome (twice the coverage in males than in females). The upper and lower green lines show the expected coverage of X-linked and Z-linked loci in a XY and ZW sex determination system, respectively. The coverage plot showing the total number of selected loci (average coverage across all individuals >3 and <400) is reported in Supplementary Fig. 2 Full size image F ST analyses confirmed our findings using the GWAS approach. Several genomic regions exhibited a high degree of genetic differentiation between males and females on LG21 (F ST > 0.5) on a background of low genome-wide differentiation (average F ST across all loci = 0.004). This pattern was consistent across the three different sliding windows used (1, 10 and 100 Kb). F ST analysis confirmed the weaker association found on LG7 using the GWAS approach. Across the three windows used, several regions consistently exceeded the set threshold, showing an average F ST value in the upper 1% of the distribution of the per window F ST values. However, the majority of the windows exceeding the threshold were located on LG21 (see Supplementary Data 3 and Supplementary Fig. 1 ). To provide further confirmation of the genomic regions associated with sex in X. hellerii , we analysed coverage information from males and females in order to identify any non-recombinant regions along chromosomes. Here, we used the X. hellerii genome v3.0.1 [47] for aligning the RAD reads, derived from a single female, the heterogametic sex in a W/Z sex chromosome system. By investigating copy number variation, we detected 18 candidate female-specific loci (mean coverage in females >7; mean coverage in males <2) (Fig. 2c , Supplementary Fig. 2 and Supplementary Data 4 ) and no male-specific loci. Again, such a pattern is compatible with female heterogamety and a W/Z sex chromosome system. We then aligned these loci to the X. maculatus genome v4.4.2 to compare the location of the sex-determination system in the two Xiphophorus species. We found that out of the total 18 female-specific loci, 16 aligned to the X. maculatus genome, 14 of which were on LG21, which is the sex linkage group (Supplementary Data 4 ). This indicates that the sex-chromosome pairs of X. hellerii and X. maculatus are homologous. We then identified potential Z-linked loci (mean coverage ratio in male/female >1.9) (Fig. 2c , Supplementary Fig. 2 and Supplementary Data 4 ). Of these, we found that 161 loci aligned to the X. maculatus genome, and the highest number of loci aligned to LG21 (54: 33.5%), followed by LG13 (27: 16.8%) and LG10 (17: 10.5%) (Supplementary Fig. 3 and Supplementary Data 4 ). Both the W-linked female-specific loci and the Z-linked male loci were found to be over-represented on LG21 (two-tailed Fisher exact test: p -value < 0.001). The occurrence of several Z-linked loci that did not align to X. maculatus LG21 could suggest the presence of autosomal modifiers. However, given the potentially high false positive rate when using such an approach, caution is needed in interpreting these findings. Taken together the GWAS, F ST and coverage analysis results show that the Rio Lancetilla population of X. hellerii , which is the paternal species in our long-term crossing experiment, has a ZW chromosome system. LG21 is the sex chromosome pair and includes a terminal non-recombining region (spanning from approximately 13 to 23 Mb) and a large (0–13 Mb) pseudoautosomal region (PAR). The boundary between the non-recombining region and the PARs was identified by a sudden drop of SNPs significantly associated with sex, as revealed by the GWAS (Fig. 2b and Supplementary Data 2 ), a pattern confirmed by the F ST (Supplementary Fig. 1 and Supplementary Data 3 ) and the coverage analysis (Supplementary Data 4 ). Despite X. maculatus having a different type of genetic sex determination, the sex chromosomes of both parental species are homologous. Introgression of parental DNA in a controlled backcrossing experiment We performed a laboratory cross, hybridisation with backcrossing, and sequenced the first and approximately 100th generation backcross individuals (sequencing statistics for each individual are provided in Supplementary Data 5 ). This crossing experiment mimicked the evolutionary scenario that has potentially given rise to two Xiphophorus fish species, X. clemenciae and X. monticolus , and in which the parental species differ in their sex chromosome systems (see refs. [26] , [33] , [36] , [37] , [43] ). Accordingly, we crossed a female Southern platyfish ( X. maculatus , genotype 2 N = 48; XX) with a male swordtail ( X. hellerii , genotype 2 N = 48; ZZ). A female F 1 fish was used for producing the first backcross with X. hellerii . Further on, female fish were selected in each backcross generation for two pigmentation phenotypes that are encoded on X. maculatus X-chromosome (LG21) close to a molecular marker, the xmrk oncogene, and mated to X. hellerii males. Not unexpectedly, the crossing of two species with opposing sex chromosomal systems produced an F 1 generation that showed severe signs of hybrid dysgenesis. In such crossing, the number of offspring that developed to adulthood was very low (usually 1–3, compared to 20–50 in the purebred parental species) and a considerable number of these were sterile (Supplementary Table 1 ). This was particularly the case for females, which carry the X. maculatus X chromosome, which was our target for selection in the long-term crossing experiment. 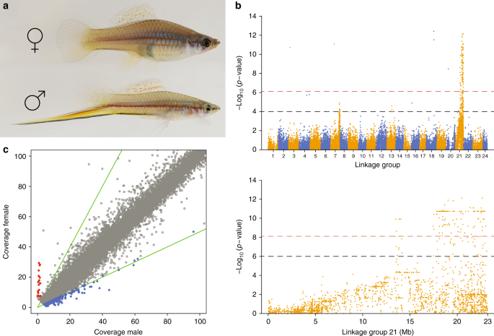Fig. 2 Sex-determination system inXiphophorus hellerii.aA male and female specimen ofX. hellerii, males are clearly distinguished by the elongated caudal fin, ‘the sword’ (Fish images by M. Schartl).bGenome-wide association analysis, where sex is set as a binary case/control variable. The 65,417 SNPs that passed quality control were used in this analysis. The Manhattan plot shows the −log10p-value (Fisher’s exact test) of each SNP across the 24X. maculatuslinkage groups (LGs). The dashed red line indicates the genome-wide significance level (p-value = 7.79e−7), while a suggestive significance (p-value = 0.001) is denoted by the dashed black line. Orange and blue colours are used to distinguish between LGs. The peak showing the strongest association is located on LG21, and is enlarged in the bottom-right section of the panel.cSequence coverage of RAD loci in female and maleX. helleriiindividuals. Each dot in the scatter plot represents the average coverage across all males (x-axis) against the average coverage across all females (y-axis) for each of the selected RAD loci. Red dots indicate potential W-linked loci (female-specific loci), while blue dots indicate loci potentially linked to the Z chromosome (twice the coverage in males than in females). The upper and lower green lines show the expected coverage of X-linked and Z-linked loci in a XY and ZW sex determination system, respectively. The coverage plot showing the total number of selected loci (average coverage across all individuals >3 and <400) is reported in Supplementary Fig.2 Conversely, those offspring from backcrosses to X. hellerii , including BC 100 , displayed full fertility and a clear-cut sex-linked inheritance of the pigmentation loci (Supplementary Table 2 ). All fish (99.7%) with these markers were females, while the fish without the selected markers were preponderantly males (91.7%). A clear enrichment of maternal alleles was observed in the BC 1 _pigm group (Fig. 3 ) as expected at LG21 (maternal/paternal allele ratio >0.9) in a genomic region close to the xmrk oncogene of X. maculatus (Fig. 3 ). In the >100 backcross generation, maternal polymorphisms were found at 476 SNPs in the BC 100 _pigm group, and at 158 SNPs in the BC 100 _wt group (Table 1 and Fig. 4 ; see the ancestry frequency calculated at each SNP in Supplementary Fig. 4 ). Notably, in the BC 100 _pigm a large block of retained maternal polymorphisms (204 SNPs) spanning approximately 10 Mb was found in the central part of LG2 (Fig. 4 ). Specifically, several loci with X. maculatus alleles were retained in the BC 100 _pigm group, which in the genome of the parental X. maculatus exclusively identify scaffolds from LG21 that are located in the region containing xmrk and the pigmentation loci. No such enrichment was seen on LG21 of the BC 100 _pigm group. Hence, this genomic region in the backcross hybrids is derived from the X. hellerii genome. Fig. 3 Parental allele ratios in the first generation backcross. Maternal and paternal allele ratios in BC 1 _wt (blue line) and BC 1 _pigm (orange line) on LG2 and LG21. The location of the melanoma gene ( Xmrk ), linked to the pigmentation genes, in LG21 is shown Full size image Table 1 Segregation patterns of the parental alleles Full size table Fig. 4 Segregation patterns of parental alleles. a Frequency of loci carrying platyfish alleles in the BC 100 _wt (blue bars) and BC 100 _pigm (orange bars) in each of the 24 linkage groups of the X. maculatus genome; b frequency of maternal alleles across linkage group 2 (LG2) Full size image To identify genomic regions in hybrid individuals that harbour X. maculatus polymorphisms, parental alleles were sorted according to a set of key criteria, sites carrying a maternal variant in at least one individual of the BC 100 generation were identified and annotated, and the ancestry frequency of each SNP was calculated. For this analysis, the region in the BC 100 _pigm showing high maternal allele density in LG2 was masked because of the hypothesized different mechanisms by which it was produced (translocation of the X. maculatus sex-determining region to an autosome of the receiving genome). After removing these sites, a total of 204 loci with maternal alleles were identified in the BC 100. Our simulations show that the number of retained X. maculatus polymorphisms is higher than expected under a neutral model of hybridisation with backcrossing ( p < 0.001; Fig. 4 ). This suggests that selection has shaped the hybrid genomes beyond LG2. By conducting a long-term evolutionary crossing experiment, we demonstrate the genomic consequences, and particularly the consequences of sex chromosome evolution, of hybridisation with backcrossing to the paternal species. This same mechanism has potentially contributed to the evolutionary history of two Xiphophorus fish species. Importantly, the parental species in this cross differ in their sex chromosome systems. We find that artificial selection for pigmentation phenotypes in backcrossed individuals results in the retention of a large, maternally derived genomic block after 100 generations (>30 years). Interestingly, this experimental design has unexpectedly promoted the formation of a new sex chromosome, and although no other known selection is imposed under our experimental conditions, there is also a higher proportion of maternal SNPs retained elsewhere in the genome than expected under a neutral model. The retention of certain X. maculatus alleles in synthetic swordtail–platyfish hybrids thus appears to be a phenomenon that occurs across a very short timescale and may be driven by a range of non-mutually exclusive forces. In the synthetic hybrid lineage, maternal ( X. maculatus ) alleles are concentrated within a region of approximately 10 Mb on LG2 after about 100 backcross generations. Such a concentration is not seen elsewhere in the genome, or in the wild-type non-selected hybrid lineage. We suggest that a combination of two proximate mechanisms may have contributed to the retention of this unexpectedly large maternal genomic block. Firstly, a mechanism likely contributing to the generation and or maintenance of this genomic pattern is a translocation event accompanied by recombination suppression. Specifically, potentially sometime during the establishment of the selected backcross line the region of LG21 known to encompass the black pigmentation locus Sd including the xmrk oncogene, the female sex-determining locus, and the red colour pattern locus Dr was translocated into the region on LG2. By imposing selection for these genes (a small region of former LG21 [46] ), the genes and the surrounding non-recombining regions on LG2 are transmitted as a large block. Second, theoretical predictions suggest that blocks of an introgressing genome are expected to be longer around selected loci [48] . Therefore, due to artificial selection of two genes, sometime during the early backcross generations a large maternally derived block encompassing the selected genes may have been maintained. We note that the higher proportion of maternal SNPs retained elsewhere in the genome may be due to the selection of fertile individuals in each backcross generation, and therefore the purging of incompatible combinations of alleles while an excess of maternal alleles are left. Given that the core of the retained genomic block originates from the X chromosome and includes the sex-determining locus (from X. maculatus ), the genomic consequences of this form of hybridisation followed by repeated backcrossing and selection appears to include the formation of a new sex chromosome. Our results strongly suggest that an X chromosome from the platyfish, X. maculatus , was introgressed into the genome of the swordtail, X. hellerii , which has a ZW sex chromosome system. After approximately 100 generations of backcrossing, the platyfish X-chromosome derived sex-determining region (X-SD) has moved to what was previously an autosomal location. While in the purebred platyfish homozygosity at the Sd region of X is required for female development, in the BC 100 heterozygosity is sufficient. Thus the recombinant neo-sex chromosome behaves like a W with a dominant effect on SD. In the backcrosses, only male X. hellerii were used, and the almost exclusive female sex of the fish expressing the selected colour loci on LG2 in the highest backcross generations show that the Z-chromosome (LG21) in X. hellerii has no male determining power. Our observation that the sex-determining region of the X was translocated to an autosome provides the first empirical evidence of a heterologous transition. Additionally, at its new chromosomal position the former X-chromosome specific region is located within a large region of retained maternal sequences, indicating that the loss of recombination accompanied the establishment of the novel W chromosome. This formation of a new sex chromosome under a hybridisation with backcrossing scenario highlights the possibility that the variation in genetic sex-determining mechanisms found in the genus Xiphophorus , which include simple male and female heterogametic systems together with more complicated situations [24] , may be contributed to by the many hybridisation events inferred among species in this genus. More specifically, this formation of a new sex chromosome provides a key target for future functional studies, and for further investigations of the Xiphophorus species thought to have arisen through hybridisation with backcrossing in the wild. For example, could this new sex chromosome play a role in reproductive isolation? And do the sex chromosomes of wild hybrids play similar roles? The X chromosome has been found to play a special role in reproductive isolation in many species, most likely due to Haldane’s rule, meiotic drive or faster evolution (‘faster X’) [49] . However, to date a definitive role for the X chromosome in reproductive isolation and speciation remains elusive in Xiphophorus . In another Xiphophorus species, Xiphophorus nezahualcoyotl, that exhibits significant hybrid ancestry, it has been indicated that the putative X chromosome has lower levels of coding and non-coding introgression than average, although reportedly not a clear outlier from other chromosomes [27] . Sex chromosome systems in closely related species of fish are generally highly variable, suggesting changes occur rapidly in these systems, and neo-sex chromosomes or novel SD regions have been reported in natural populations [50] , [51] , [52] , [53] , [54] , [55] . More broadly, further studies of hybridisation in this genus are imperative for fully understanding the genomic and adaptive consequences of the process, including at different time scales. Importantly, recent advances have been made in the development and application of genomic methods for detecting hybridisation and inferring individual ancestries [56] , [57] , [58] . Indeed, fine-scale signals of hybridisation can be detected using genomic analyses that allow the identification of introgressed genes and gene combinations which may be important in adaptation (e.g. refs. [59] , [60] , [61] ). Also, long-read de novo assemblies of various species allow more refined measures of genomic introgression events, a necessary measure to develop evolutionary theories of molecular mechanisms. Broadly, research to date suggests that hybridisation can be a mechanism for co-opting functional elements from another genome [61] , [62] . For instance, modern humans carry genomic regions derived from Neanderthal ancestors including loci involved in skin and hair phenotypes suggested to be adaptive for humans migrating to non-African environments [61] , [62] . Importantly, previous studies have suggested that the rate of hybrid genome stabilisation varies across taxa and is dependent on demographic differences, selection or strong genetic drift [57] . In rare and extreme cases, whole genome hybridisations can alter the course of major traits such as meiosis [38] . In the current study, by using an experimental backcross for over 100 generations we could directly observe the genomic consequences of hybridisation with backcrossing. Importantly this was done with two parental species with different sex (determining) chromosome systems, and where we strongly selected for distinct phenotypes. It is likely that a combination of different processes drove the observed genomic outcomes, including exogenous selection (i.e. artificial selection for the pigmentation phenotype and female sex), and endogenous selection such as gene–gene interactions. Further, the genomic patterns observed here could have come about through a number of different scenarios that require future investigation. For instance, the patterns may reflect the potential for a connection between chromosomal organisation and adaptive evolution in this system. Alternatively, and potentially equally parsimoniously, the translocation event may have also been neutral. Recombination suppression associated with chromosomal rearrangement can promote local adaptation and the accumulation of genetic incompatibilities between species (reviewed in refs. [63] , [64] ). In Helianthus sunflowers, where large linkage blocks appearing to resist recombination were observed in both experimental and ancient hybrids, gene interactions were invoked as the most likely explanation for the observed concordance in genomic pattern [65] . In another more recent study where introgression and local adaptation in two poplar species were investigated using fine-scale genomic techniques, admixed individuals of one species harbour a telomeric region on one chromosome which had introgressed from the other species, and this region was found to contain several candidate genes for local adaptation [59] . Interestingly, a paralogous block of genes on another chromosome showed no signs of introgression or signatures of selection [59] . Natural hybridisation between several species in the genus Xiphophorus has been inferred and has reportedly occurred across different timescales, including contemporary and more ancient events [27] , [34] , [36] , [37] , [39] , suggesting hybridisation, such as the scenario investigated in our study, may be a key contributor to the evolutionary history of this group of fishes. Sex determination in Xiphophorus hellerii A total of 30 female and 30 male X. hellerii individuals from the same strain (origin Rio Lancetilla), which were also used for the backcrossing experiment, were genotyped to identify sex-related markers, and thus characterize the sex determination system of this swordtail species strain. Sequencing and data filtering Genomic DNA was extracted from fin clips using standard phenol–chloroform extraction [66] , followed by RNase treatment. DNA quality of each sample was assessed by agarose gel electrophoresis and quantified using a Qubit v2.0 fluorometer (Life Technologies, Darmstadt, Germany). Approximately 100 ng of DNA template of each sample was used to construct a single quaddRAD [67] library (PstI and MspI were used as rare and frequent restriction enzymes, respectively), size selected from 450 to 550 bp using a Pippin Prep platform (Sage Sciences, Beverly, USA) and paired-end sequenced in an Illumina HiSeq2500 (rapid run mode, 2 × 151 cycles). The raw fastq files obtained from one Illumina lane (NCBI’s SRA database, accession no. PRJNA493969) were first processed using the clone_filter module implemented in the Stacks v1.46 [68] , [69] package to identify and remove duplicate reads. The retained sequence data, stripped of the four random bases at the 5′ end of each paired read, was then separated by the dual index inner barcodes using the Stacks’ process_radtags script (option: –inline_inline ) with no quality filters applied. Next, the sequences were processed by the dDocent v2.2.25 pipeline [70] , with default parameters, in order to get the individuals’ genotypes. For this RAD data set, the dDocent pipeline was preferred to Stacks because of its superior ability to deal with paired-end reads when calling genotypes. Briefly, dDocent calls Trimmomatic v0.36 [71] , bwa v0.7.15 [72] and Freebayes v1.1.0 [73] to respectively quality control the raw reads, align the filtered sequences to the reference genome and infer individuals’ genotypes at polymorphic loci. Trimmomatic was used to remove bases with a quality score <20 from the beginning and end of reads, and additionally trim bases with an average quality score <10 in a sliding 5 bp window. The ‘mem’ algorithm implemented in bwa was applied setting the match score value (-A) to 1, the penalty for a mismatch (-B) to 4 and the gap penalty (-O) to 6. Freebayes was used to call genotypes setting a minimum mapping and base quality score to 10. Sequence variation analysis: filtering and GWAS of sex in X. hellerii The raw VCF variant file was obtained by setting the X. maculatus v4.4.2 as the reference genome [46] . In this version of the X. maculatus genome, the original scaffolds [43] were tiled along a dense genetic map to create chromosome-length genome assemblies. The VCF file was filtered using VCFtools v0.1.15 [74] to retain loci present in a minimum of 80% of the individuals and having mapping quality (MQ) > 30. Further stringent filtering was applied using the dDocent_filters script ( http://ddocent.com/filtering/ ) that relies on both VCFtools and the vcffilter module in the vcflib package ( https://github.com/vcflib/ ). 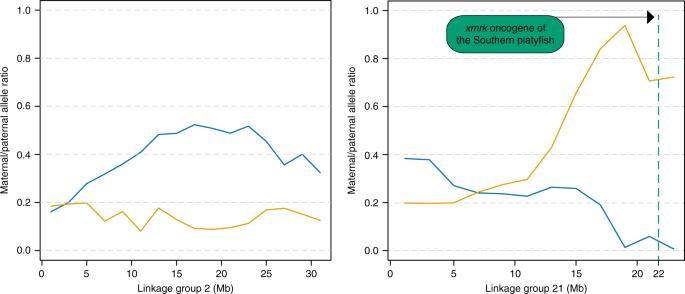Fig. 3 Parental allele ratios in the first generation backcross. Maternal and paternal allele ratios in BC1_wt (blue line) and BC1_pigm (orange line) on LG2 and LG21. The location of the melanoma gene (Xmrk), linked to the pigmentation genes, in LG21 is shown 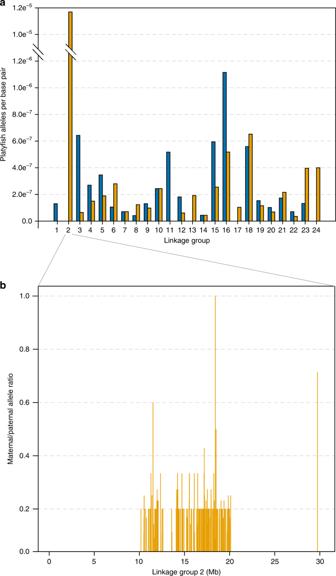Fig. 4 Segregation patterns of parental alleles.aFrequency of loci carrying platyfish alleles in the BC100_wt (blue bars) and BC100_pigm (orange bars) in each of the 24 linkage groups of theX. maculatusgenome;bfrequency of maternal alleles across linkage group 2 (LG2) A total of 65,417 SNPs passed the quality control applied and were used for the GWAS and the F ST analyses (the full set of filters, and the number of sites removed at each step, are reported in Supplementary Table 3 ; the individuals’ genotypes were deposited into the Dryad Data Repository: https://doi.org/10.5061/dryad.7h54h66 ). The final VCF file was used to perform a standard genome-wide association analysis using PLINK v1.90b4.9 [75] setting sex as the binary case/control variable. The −log 10 p -value (obtained with a Fisher’s exact test) of each SNP was shown as a function of genomic position on the 24 X. maculatus LGs [46] in a Manhattan plot constructed with the R package qqman v0.1.4 [76] . The threshold for genome-wide significance was set at a p -value = 7.64e −7 after Bonferroni correction for multiple comparisons (0.05/65,417 variants). To identify highly divergent, potential candidate sex-chromosome regions using an additional line of investigation, the program VCFtools was used to calculate F ST -values between males and females across different non-overlapping sliding windows (1, 10 and 100 Kb). As a suggestive threshold for significance, we used the upper 1% percentile distribution of the per window F ST values (1 Kb window: F ST = 0.184; 1 Kb window: F ST = 0.181; 1 Kb window: F ST = 0.157). Coverage analysis to identify sex association in X. hellerii As an alternative and independent approach to identify and verify potential sex-associated SNPs, we analysed mapped sequence coverage information from X. hellerii males and females to identify loci located in the non-recombining and recombination restricted regions of the sex chromosomes. We first created a set of reference loci using the ustacks module of the Stacks package in default mode, but setting the minimum depth of coverage required to create a stack (-m) to 5. As a reference for aligning the RAD loci, we used the X. hellerii genome v3.0.1 (NCBI accession number: GCA_001443345.1) [47] that is derived from a single female, strain Sarabia, from the Xiphophorus Genetic Stock Center (TX, USA). Existing evidence suggested that the female is the heterogametic sex in this species; therefore, because the genome of X. hellerii was generated using a single female individual, using the X. hellerii genome would allow us to recover a higher number of W-linked loci than using the X. maculatus genome. We used this approach to confirm the findings of the statistically more robust GWAS approach, and possibly to identify specific X. hellerii sex-determining regions (e.g. autosomal modifiers). The total 70,763 loci, extracted from the Stacks’ catalogue formatted in fasta format (deposited into the Dryad Data Repository: https://doi.org/10.5061/dryad.7h54h66 ), were used as a reference for the alignment of the sequence set of each sample carried out with Bowtie2 v2.3.0 [77] in ‘--very-sensitive’ mode. To avoid redundant information, only one of the paired loci was retained to serve as a reference. Next, raw coverage values—i.e. the number of reads mapping to each locus—were extracted from each individual mapping file using SAMtools v1.2.1 [78] idxstats and normalized using the Median Ratio Normalization (MRN) function implemented in DESeq2 v1.8.1 [79] . We then calculated the mean coverage for each locus (including males and females), but first removed loci with coverage below 3 and above 400 because they most likely indicate mapping errors and repetitive elements, respectively (the number of loci was reduced to 29,444 after the coverage filters were applied). We assumed a ZW sex-determination system is operating in this system, given the results from our sequence variation analysis (see the previous paragraph), and from the filtered coverage data set we selected (1) potentially W-linked female-specific loci and (2) Z-linked loci. According to expectations, W-linked loci should be present only in females, the heterogametic sex, so we applied coverage filters to satisfy this condition (mean coverage in females >7; mean coverage in males <2). On the other hand, the Z-linked loci are expected to be present in both sexes, but they should have twice the coverage in males than in females, as they have two copies of the Z chromosome (coverage filter to identify these loci: mean coverage ratio in male/female >1.9). We note that this type of filtering criteria is dependent on the sequencing depth of coverage used in the experiment, and the use of these arbitrary filters means the results should be interpreted with caution. However, the main purpose of the coverage analysis was to confirm the results of the GWAS analysis. Finally, we used a two-tailed Fisher’s exact test to test for over-representation of these candidate sex-chromosome loci in the X. maculatus LGs that were associated with sex (SNP analysis). Synthetic hybrids: laboratory cross experiment Laboratory crosses were conducted which mimic the hybridisation with backcrossing evolutionary scenario that has potentially given rise to at least two Xiphophorus fish species, and may have contributed to the ancestry of other taxa. We sampled both first generation and approximately 100th generation backcrossed individuals that had been artificially selected for two pigmentation phenotypes. We note that all sampled backcross generations were raised under the same standard laboratory conditions, therefore excluding any environmental effects. In these laboratory crosses, one parental species is X. maculatus , where the strain Jp163A (origin Rio Jamapa) was used, which is also the same strain from which the reference genome was produced [43] . This strain has been kept as a brother–sister mating line for more than 100 generations. The other parental species used in the laboratory crosses is X. hellerii . The stock is derived from fish collected from the Rio Lancetilla and has been kept for over 50 years in closed colony breeding. The X. hellerii stock has been through several bottlenecks (due to the breakdown of the stock) where only a handful of fish or even a single pair was used to regenerate the stock. Both parental species are representatives of the two clades that were earlier shown to have been involved in the initial hybridisation event generating X. clemenciae and X. monticolus [33] , [36] , [37] . The first generation hybrid cross was between a female X. maculatus and a male X. hellerii . Next, a backcross was made between an F 1 female, carrying the pigmentation phenotypes intended for selection and an X. hellerii male. Females were then selected for each successive backcross according to the two colour markers. One is the erythrophore pigmentation pattern dorsal red , Dr , which causes a dark red colouration of the dorsal fin and in hybrids extends from there over the whole body and the unpaired fins. The second pattern is caused by the closely linked macromelanophore pattern locus spotted dorsal , Sd . It is expressed as jet-black pigmentation spots at the base of the dorsal fin in purebred X. maculatus . In the genetic background of X. hellerii , the macromelanophores cover the whole dorsal fin, and from there invade the dorsal and caudal body compartment of the fish. As an effect of the Sd locus component, xmrk oncogene [74] , the macromelanophore pattern in the genetic background of X. hellerii is enhanced to melanotic hyperpigmentation that can progress to malignant melanoma (for an overview of the pigmentation genetics of platyfish/swordtail hybrids, see ref. [40] ). Dr and Sd/xmrk are closely linked on the X-chromosome of the platyfish corresponding to linkage group 21 [43] , [46] . In the serial backcross experiment, each generation consists of 50% fish with and 50% without the chromosome region where both genes are located, designated as ‘pigm’ or ‘wt’ group. Selecting fish with the two linked colour markers for breeding mimics natural selection for a certain phenotype. Therefore, we expect fish with the pigmentation phenotype to carry the parental platyfish genetic region of the X-chromosome. Backcrossing was continued in this fashion for at least 100 generations (more than 30 years of laboratory crosses have been performed, counting was terminated after backcross 50 and on average three backcross generations were produced per year). For the approximate 100th generation backcross offspring, we expect fish carrying the pigmentation genes (further on referred to as BC 100 _pigm) to be enriched for genetic markers of platyfish LG21. By contrast, segregants not carrying the colour genes (wild type pigmented, further on referred to as BC 100 _wt) should not be enriched for platyfish sequences of this region of the genome. Sequencing, filtering and genotype calling Genomic DNA was extracted from pooled organs (brain, eyes, gills, liver, spleen, kidney) of the two parental species (two males and two female individuals each for X. maculatus and X. hellerii ), four F 1 females, 16 first generation backcross individuals and 18 individuals generated after about 100 backcross generations. DNA extraction was carried out using the standard phenol–chloroform extraction [66] . The DNA quality of each sample was determined by agarose gel electrophoresis and quantified using a Qubit v2.0 fluorometer. Approximately 300 ng of DNA template of each sample was used to construct double-digest restriction site-associated DNA (ddRAD) [80] libraries following the modifications introduced in ref. [81] . DNA digestion was carried out using the restriction enzymes PstI (rare cutter) and MspI (frequent cutter). A single ddRAD library containing 46 barcoded individuals (see Supplementary Data 3 for details) was constructed, size selected from 360 to 430 bp using a Pippin Prep system and single-end sequenced in an Illumina HiSeq2500 using rapid run mode with 151 cycles (raw reads were deposited in the NCBI’s SRA database, accession no. PRJNA493969). The process_radtags script implemented in the Stacks package was used for individual demultiplexing and for filtering erroneous and low-quality reads (options: -c –q). After this process, an average of 2.95 million ( X. maculatus ) and 2.08 million ( X. hellerii ) sequences were obtained for the parents; an average of 3.05, 1.91 and 2.34 million sequences were obtained for the F 1 , BC 1 and BC 100 individuals, respectively (see Supplementary Data 3 ). The sequence length of each read was 146 bp after removing its 5-bp barcode. Filtered reads were individually aligned to the anchored version of the X. maculatus genome [46] using Bowtie2 with default end-to-end mode. SAMtools was then used to filter the mapping result by retaining only sites with high quality score (MQ ≥ 30). Loci construction and genotype calling were performed using the Stacks’ ref_map.pl pipeline requiring a minimum of five reads (- m 5) to form a locus and calling genotypes at a 5% significance level using the bounded error model (upper bound of 0.05). The allelic variants (SNPs) were exported in VCF format using the Stacks’ populations module. Sorting of parental alleles in the laboratory cross dataset An in-house Perl script was used to identify the subset of sites fixed for alternative alleles in the two parental species ( X. maculatus and X. hellerii ) of the laboratory cross following these criteria: (1) the individuals’ genotypes are homozygous within each parental species, but they have different allelic variants; (2) the sites selected previously are heterozygous including both parentals’ allelic variants in F 1 individuals; (3) at these sites, all BC 1 and BC 100 individuals have at least one paternal ( X. hellerii ) allele. After these filtering steps, we obtained a total of 34,632 SNPs (the individuals’ genotypes were deposited into the Dryad Data Repository: https://doi.org/10.5061/dryad.7h54h66 ). Tests for excess ancestry As we focused on SNPs fixed between the parental species (see above), each SNP was fully informative about ancestry. Thus, we were able to directly calculate the frequency of platyfish ancestry in the BC 100 lines. We then used a stochastic simulation to develop null expectations for the frequency of platyfish ancestry expected in the absence of selection after 100 generations of backcrossing. We sampled platyfish ancestry frequencies each generation stochastically as y t = binomial( p t−1 * 0.5, 2 N ) and then set p t = y t /2 N . Here, y t is the number of platyfish alleles in the sample of N diploid hybrid fish and p t and p t−1 are the ancestry frequencies in the current and previous generation, respectively. The expectation for the binomial is reduced by half each generation as the BC line is backcrossed to X. hellerii . Using this iterative process and starting from p 0 = 0.5 (F 1 s), we simulated expectations for 100 generations of backcrossing with N = 10 or 15 hybrid fish per generation (conservative estimates of the average number of fish used to maintain the line over time). We repeated this procedure 10,000 times. In all cases, we found expected platyfish ancestry at generation 100 of p 100 = 0. Ethical statement All animals were kept and sampled in accordance with the applicable EU and national German legislation governing animal experimentation. In particular, all experimental protocols were approved through an authorization (568/300-1870/13) of the Veterinary Office of the District Government of Lower Franconia, Germany, in accordance with the German Animal Protection Law (TierSchG).